Phase and structure engineering of copper tin heterostructures for efficient electrochemical carbon dioxide reduction While engineering the phase and structure of electrocatalysts could regulate the performance of many typical electrochemical processes, its importance to the carbon dioxide electroreduction has been largely unexplored. Herein, a series of phase and structure engineered copper-tin dioxide catalysts have been created and thoroughly exploited for the carbon dioxide electroreduction to correlate performance with their unique structures and phases. The copper oxide/hollow tin dioxide heterostructure catalyst exhibits promising performance, which can tune the products from carbon monoxide to formic acid at high faradaic efficiency by simply changing the electrolysis potentials from −0.7 V RHE to −1.0 V RHE . The excellent performance is attributed to the abundant copper/tin dioxide interfaces involved in the copper oxide/hollow tin dioxide heterostructure during the electrochemical process, decreasing the reaction free-energies for the formation of COOH* species. Our work reported herein emphasizes the importance of phase and structure modulating of catalysts for enhancing electrochemical CO 2 reduction and beyond. The increased CO 2 level in the atmosphere has caused many climatic concerns, such as global warming, melting glaciers, and more disastrous weather [1] . The conversion of CO 2 into renewable energy sources has attracted extensive attention; this conversion not only decreases the CO 2 concentration in the atmosphere but also stores renewable energy [2] , [3] , [4] , [5] . Recently, the electroreduction of CO 2 has attracted particular attention [5] , [6] , mainly due to its feasible operating conditions and the potential of sustainable direct integration with renewable resources. Many studies have reported the electrochemical CO 2 reduction reaction (CO 2 RR) by using different catalysts [6] , [7] . For example, noble catalysts, such as Au [8] , [9] , Ag [10] , [11] , and Pd [12] , are generally reported to reduce CO 2 into CO, whereas main group metals In [13] , Sn [14] , Pb [15] , and Bi [16] favor the generation of formic acid (HCOOH) during the CO 2 RR. Unlike noble metal and main group metal catalysts, Cu is active to electroreduce CO 2 into hydrocarbons or oxygenates [17] , [18] , [19] , but it also generates common products, such as CO, HCOO − and H 2 [20] , [21] . Owing to the unique behavior of Cu in the CO 2 RR, substantial research efforts have been devoted to improve the activity and selectivity of Cu catalysts for the CO 2 RR [22] , [23] . Nevertheless, the achieved faradaic efficiency (FE) for the useful products is unsatisfactory and usually <40%. To this end, increasingly more researchers focus on combining other metals with Cu to achieve bimetallic Cu-based catalysts [13] , [24] , which could bring extra synergistic effects or stabilize the reaction intermediates to improve the activity and selectivity of the CO 2 RR [25] , [26] , [27] , [28] . Recently, relevant works, such as the synthesis of CuAu [25] , CuPd [26] , and CuSn [27] , [28] bimetallic catalysts, etc. have been intensively reported, showing the enhanced performance for the CO 2 RR [25] , [26] , [27] , [28] . However, it should be pointed out that, while the majority of these previous studies focus on improving the CO 2 RR selectivity for only one product, the selectivity for different useful products at high levels cannot be tuned. In addition, most of these reports are limited to studying the composition (ratio of two metals) effect for the CO 2 RR, while the structure and phase effects of bimetallic catalysts on the CO 2 RR are largely unexplored. It is well known that the bimetallic-based catalyst structures (e.g., core–shell structures, heterostructures, alloying structures, etc.) or phases (e.g., metal/metal phases, metal/oxide phases, metal/sulfide phases, etc.) usually have significant influences on their electrochemical performance [29] . Such observations have been demonstrated in several electrochemical processes, such as the hydrogen evolution reaction (HER) and the oxygen reduction reaction [30] , [31] , [32] , while limited studies have revealed the structure and phase effects on the CO 2 RR. Herein, by taking advantage of the intrinsic chemical reactivity differences of the bimetallic components, we successfully develop three distinct Cu–SnO 2 bimetallic catalysts with different structures and phases: the CuO/hollow SnO 2 heterostructure of CuSn nanoparticles (NPs)/C-A, the Cu 41 Sn 11 @SnO 2 core–shell structure of CuSn NPs/C-H, and the Cu NPs/hollow SnO 2 Janus structure of CuSn NPs/C-AH through a simple yet efficient post-annealing treatment of CuSn core–shell NPs at controlled conditions. These Cu–SnO 2 bimetallic catalysts are thoroughly exploited for the electrochemical CO 2 RR, and the CO 2 RR performance is correlated with their unique structures and phases. This reveals that the optimized CuSn NPs/C-A exhibits promising activity and selectivity for the electrochemical CO 2 RR, which can tune the product from CO to HCOOH at high FE values by simply changing the electrolysis potential from −0.7 to −1.0 V RHE . Moreover, it also exhibits the highest CO 2 RR activity in all the Cu–SnO 2 bimetallic catalysts, where the partial current densities of CO at −0.7 V RHE are 5.9 and 5.3 times higher and of HCOOH at −1.0 V RHE are 33.2 and 3.4 times higher than those of the individual Cu NPs/C and SnO 2 nanoshell/C (SnO 2 NSL/C), respectively. We attribute the excellent CO 2 RR performance to its abundant Cu/SnO 2 interfaces involved in the CuO/hollow SnO 2 heterostructure during the electrochemical process, which decrease the reaction free-energies (Δ G ) for the formation of COOH* species. Furthermore, under a long-term durability test, these Cu–SnO 2 bimetallic catalysts can endure at least 10 h with small activity and selectivity decays. Preparation and characterization of CuSn NPs The CuSn NPs were obtained via the co-reduction of copper (II) acetylacetonate (Cu(acac) 2 ), and dibutyltin bis(2,4-pentanedionate) (C 18 H 32 O 4 Sn) at 180 °C for 3 h with ascorbic acid (AA) as the reducing agent and oleylamine (OAm) as the solvent and surfactant. Transmission electron microscopy (TEM) (Fig. 1a ) and high-angle annular dark-field scanning TEM (HAADF-STEM) images (Fig. 1b ) clearly show that the CuSn NPs are highly dispersive. The diameter of the CuSn NPs was measured to be 23.0 ± 3.5 nm (Supplementary Fig. 1 ). The Cu/Sn ratio of the CuSn NPs was determined to be 80.7/19.3 by scanning electron microscopy energy-dispersive X-ray spectroscopy (SEM-EDS) (Supplementary Fig. 2 ). Powder X-ray diffraction (XRD) (Fig. 1c ) was carried out to study the phase of the CuSn NPs; the diffraction peaks are perfectly indexed to face-centered cubic Cu, suggesting that the component of Sn are likely amorphous in CuSn NPs. The X-ray photoelectron spectroscopy (XPS) pattern was further carried out to confirm the surface environment of the CuSn NPs, where the Sn 3d 5/2 and 3d 3/2 peaks of CuSn NPs are located at 486.6 and 495.0 eV, respectively, which can be assigned to the 3d 5/2 and 3d 3/2 peaks of Sn 4+ (Fig. 1d ) [28] , confirming that the Sn species in CuSn NPs is present in the form of amorphous SnO 2 . To further investigate the distribution of amorphous SnO 2 in CuSn NPs, high-resolution TEM (HRTEM) for a single CuSn NP was carried out. As shown in Fig. 1e , it is obvious that there is an amorphous SnO 2 shell surrounding the crystalline Cu core. 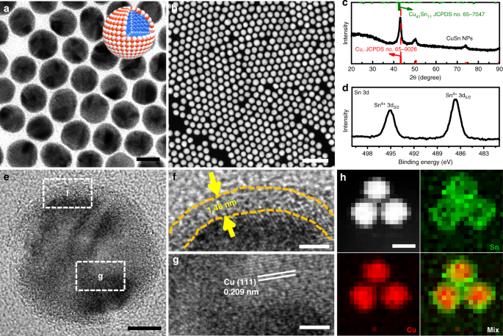Fig. 1 Structure and phase characterization of CuSn NPs.aTransmission electron microscopic (TEM) image and atom model,bhigh-angle annular dark-field scanning TEM (HAADF-STEM) image,cX-ray diffraction (XRD) pattern, anddSn 3d X-ray photoelectron spectroscopy (XPS) pattern of CuSn NPs.eHigh-resolution TEM (HRTEM) image andf,gthe magnified regions ineof CuSn NPs.hHAADF-STEM and energy-dispersive X-ray spectroscopy (EDS) elemental mapping images of CuSn NPs. Scale bars, 2 nm inf,g, 5 nm ine, 20 nm ina,h, 100 nm inb. Red, blue, and white spheres in the model represent O, Cu, and Sn atoms, respectively Figure 1f, g display the magnified images recorded from regions f and g marked in Fig. 1e , where the thickness of amorphous SnO 2 shell is approximately 1.48 nm, consistent with the HAADF-STEM line scan result of 1.43 nm (Supplementary Fig. 3 ). The interplanar spacing of the lattice fringe was measured to be 0.209 nm, consistent with the (111) plane of metallic Cu (Fig. 1g ). The distributions of Sn and Cu in CuSn NPs were further confirmed by HAADF-STEM EDS elemental mappings (Fig. 1h ), where Cu is limited to the core of the CuSn NPs, while Sn surrounds the Cu core. Hence, we can conclude that the prepared CuSn NPs have a core–shell structure with metallic Cu cores and amorphous SnO 2 shells. Fig. 1 Structure and phase characterization of CuSn NPs. a Transmission electron microscopic (TEM) image and atom model, b high-angle annular dark-field scanning TEM (HAADF-STEM) image, c X-ray diffraction (XRD) pattern, and d Sn 3d X-ray photoelectron spectroscopy (XPS) pattern of CuSn NPs. e High-resolution TEM (HRTEM) image and f , g the magnified regions in e of CuSn NPs. h HAADF-STEM and energy-dispersive X-ray spectroscopy (EDS) elemental mapping images of CuSn NPs. Scale bars, 2 nm in f , g , 5 nm in e , 20 nm in a , h , 100 nm in b . Red, blue, and white spheres in the model represent O, Cu, and Sn atoms, respectively Full size image Preparation and characterization of CuSn NPs/C-A, CuSn NPs/C-H, and CuSn NPs/C-AH Considering that the chemical reactivities of SnO 2 and Cu are quite different, the thermal annealing treatment is expected to be effective to induce phase and structure changes of the pristine CuSn NPs. We thus focus on the phase and structure engineering of CuSn NPs through annealing. To this end, the pristine core–shell CuSn NPs were loaded on a carbon (C, VC-X72) by sonication, denoted as CuSn NPs/C. The core–shell CuSn NPs are highly dispersive on C, without shape, size, phase, and composition changes after the sonication process (Supplementary Fig. 4 ). The CuSn NPs/C was then annealed at three controlled conditions. The CuSn NPs/C samples treated at 250 °C for 1 h in air and H 2 /N 2 (5/95) were denoted as CuSn NPs/C-A and CuSn NPs/C-H, respectively. The CuSn NPs/C-A sample was further annealed in H 2 /N 2 (5/95) at 250 °C for another 1 h, which was denoted as CuSn NPs/C-AH. As shown in Supplementary Fig. 5 , the EDS results reveal that the Cu/Sn ratios in CuSn NPs/C-A, CuSn NPs/C-H, and CuSn NPs/C-AH are 80.3/19.7, 79.3/20.7, and 79.2/20.8, respectively, suggesting that the thermal annealing treatment hardly induced composition changes. XRD was further carried out to analyze the structures after different annealing treatments. It is confirmed that the primary diffraction peaks of Cu largely decreased in the CuSn NPs/C-A with the appearance of distinct diffraction peaks of CuO (Fig. 2a ), suggesting that the phase of CuSn NPs/C-A was mainly transformed into CuO after annealing in air. As presented in Supplementary Fig. 6 , the CuSn NPs/C-H was transformed into the Cu 41 Sn 11 alloy, as observed in the enlarged XRD pattern between 37.0° and 47.0°. By further reannealing the CuSn NPs/C-A at 250 °C for 1 h in H 2 /N 2 (5/95) (CuSn NPs/C-AH), the CuO phase was transformed into metallic Cu. It is worth mentioning that the diffraction peaks of SnO 2 do not appear throughout the different annealing treatments, suggesting that such annealing treatment cannot crystallize the amorphous SnO 2 . Fig. 2 Structure and phase characterizations of CuSn NPs/C with controlled annealing treatment. a X-ray diffraction (XRD) patterns and inset transmission electron microscopic (TEM) images of a I CuSn NPs/C-A, a II CuSn NPs/C-H, and a III CuSn NPs/C-AH. b , d , f High-angle annular dark-field scanning TEM (HAADF-STEM) images and atom models and c , e , g HAADF-STEM images and energy-dispersive X-ray spectroscopy (EDS) elemental mappings of b , c CuSn NPs/C-A, d , e CuSn NPs/C-H, and f , g CuSn NPs/C-AH. Scale bars, 50 nm in b , d , f , 20 nm in a I – a III , c , e , g . Red, blue, and white spheres in the models represent O, Cu, and Sn atoms, respectively Full size image Besides the phase structure, the chemical states of CuSn NPs/C, CuSn NPs/C-A, CuSn NPs/C-H, and CuSn NPs/C-AH were further investigated by XPS and Auger spectra. Supplementary Fig. 7a shows the XPS pattern of Cu 2p, in which the peaks located at 952.2 and 932.3 eV belong to Cu 0,1+ species, whereas the peaks at 953.8 and 933.8 eV belong to Cu 2+ species [28] . The Cu in the initial CuSn NPs/C is in both Cu 0,1+ and Cu 2+ states. By being heated in air or H 2 /N 2 (5/95), Cu 0,1+ species in CuSn NPs/C-A disappeared, while the proportion of the Cu 0,1+ species increased in CuSn NPs/C-H. After reannealing the CuSn NPs/C-A at 250 °C in H 2 /N 2 (5/95) for another 1 h, Cu 0,1+ species reappeared in the CuSn NPs/C-AH. The Auger spectra of Cu L 3 M 45 M 45 was further carried out to distinguish the Cu 0 and Cu 1+ in these catalysts (Supplementary Fig. 8 ). In general, the characteristic peak of Cu 0 for Cu L 3 M 45 M 45 is located from 918.2 to 918.6 eV, whereas for Cu 1+ is between 916.0 and 916.4 eV and the peak for the standard Cu 2+ is from 917.6 to 917.8 eV [33] . The CuSn NPs/C-A shows a peak at 917.6 eV, confirming that there is Cu 2+ in the CuSn NPs/C-A. The CuSn NPs/C-H and CuSn NPs/C-AH all have peaks at 916.8 eV and 918.4 eV, suggesting that both Cu 0 and Cu 1+ are present in the CuSn NPs/C-H and CuSn NPs/C-AH. The binding energy of Sn 3d for these catalysts was also explored (Supplementary Fig. 7b ); the chemical state of Sn for all catalysts was mainly SnO 2 , while the binding energy of Sn in CuSn NPs/C-H and CuSn NPs/C-AH shifted to the high level of 487.0 and 486.9 eV compared to the initial CuSn NPs/C and CuSn NPs/C-A (486.6 eV), likely due to the charge transfer of SnO 2 by the reduction of H 2 . Therefore, we can conclude that the phase of CuSn NPs/C has been readily tuned by thermal annealing in controlled conditions. The electron microscopy characterizations were further utilized for investigating the structure change of CuSn NPs/C after thermal annealing at different conditions. Fig. 2a I , b show the TEM and STEM images of CuSn NPs/C-A. Interestingly, the initial solid CuSn NPs are transformed into hollow structures, with the size increasing to 26.5 ± 3.5 nm (Supplementary Fig. 9a-b ). The HAADF elemental mappings further reveal that the Sn matches well with the hollow shell accompanied by Cu on its surface (Fig. 2c ), indicating that the interior Cu diffuses outside to adhere to the hollow SnO 2 shell due to the different diffusion rates of Cu and Sn at the core/shell boundary under the annealing treatment in air [34] . The HRTEM image of CuSn NPs/C-A further shows that the lattice fringe of the section adhering on the SnO 2 shell is 0.251 nm, which is the (−111) plane of CuO (Supplementary Fig. 10a, b ). Hence, the CuSn NPs/C-A has evolved into a CuO/hollow SnO 2 heterostructure. In contrast, the structure of CuSn NPs/C-H is largely maintained compared to the initial CuSn NPs/C (Fig. 2a II , d, e and Supplementary Fig. 9c, d ), while the interplanar spacing of the core of CuSn NPs/C-H is 0.212 nm, which is the (660) plane of intermetallic Cu 41 Sn 11 (Supplementary Fig. 10c, d ), revealing that the CuSn NPs/C-H has a core–shell structure. Impressively, after reannealing the CuSn NPs/C-A at 250 °C in H 2 /N 2 (5/95) for another 1 h, H 2 transformed CuO into metallic Cu conjoined with the hollow SnO 2 shell to form a Janus structure with the increased size of 32.5 ± 4.5 nm (Fig. 2a III , f and Supplementary Fig. 9e, f ). The HRTEM and HAADF elemental mappings further confirm the Janus structure of CuSn NPs/C-AH, with the Cu NP as one side and the hollow SnO 2 as the other side (Fig. 2g and Supplementary Fig. 10e, f ). Therefore, it can be concluded that, after the phase and structure engineering by the simple thermal annealing treatment in controlled conditions, we have successfully transformed the initial core–shell CuSn NPs into three distinct catalysts with different phases and structures: the CuO/hollow SnO 2 heterostructure of CuSn NPs/C-A, the Cu 41 Sn 11 @SnO 2 core–shell structure of CuSn NPs/C-H, and the Cu NPs/hollow SnO 2 Janus structure of CuSn NPs/C-AH. All the structures are presented by their corresponding models in the inset in Fig. 2b, d, f . CO 2 RR performances of CuSn NPs/C-A, CuSn NPs/C-H, and CuSn NPs/C-AH Considering that Cu and Sn are believed to be the active components in the CO 2 RR [14] , [17] , [18] , [19] , [20] , [21] , the structure and phase effect of the CuSn NPs/C on the CO 2 RR deserves further investigation. To this end, the CO 2 RR performances of the CuSn NPs/C-A, CuSn NPs/C-H, and CuSn NPs/C-AH were fully evaluated in 0.1 M KHCO 3 (Fig. 3 ). To reveal the bimetallic effect, the Cu NPs/C and SnO 2 NSL/C were prepared as references via a solvothermal method and chemical etching of CuSn NPs/C-A, respectively (Supplementary Fig. 11 - 12 ). The CO 2 RR performance was measured by the chronoamperometry method under different potentials (Supplementary Fig. 13 ). The products in gas and liquid phase were analyzed via gas chromatography (GC) and nuclear magnetic resonance (NMR), respectively (Supplementary Fig. 14 - 15 ). Figure 3a shows the polarization curves of CO 2 RR using linear sweeping voltammetric methods at 5 mV s −1 . 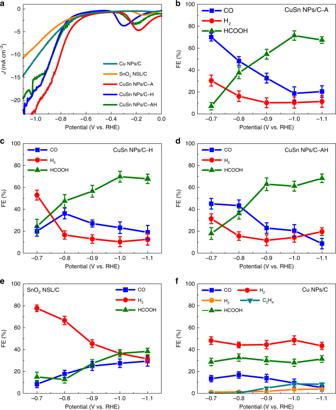Fig. 3 Electrochemical CO2reduction performance of various Cu–SnO2catalysts, Cu NPs/C and SnO2NSL/C.aLinear sweeping voltammetric curves of electrochemical CO2reduction measured in 0.1 M KHCO3for different catalysts. Scan rate: 5 mV s−1. Reduction potential-dependent faradaic efficiencies (FEs) of H2, CO, and HCOOH forbCuSn NPs/C-A,cCuSn NPs/C-H,dCuSn NPs/C-AH,eSnO2NSL/C, andfCu NPs/C Compared to the SnO 2 NSL/C and Cu NPs/C, all the Cu–SnO 2 bimetallic catalysts with different phases and structures exhibit relative high activity from −0.7 to −1.1 V RHE , suggesting that the combination of Cu and Sn enhances the electrocatalytic response. Figure 3b, f show potential-dependent FEs of the major products for CO 2 RR by using different catalysts. The electrocatalytic process mainly produces H 2 , CO, and HCOOH from −0.7 to −1.1 V RHE as well as CH 4 and C 2 H 4 at −1.0 and −1.1 V RHE for all catalysts except SnO 2 NSL/C (Supplementary Fig. 16 ). The Cu–SnO 2 bimetallic catalysts exhibit lower FE H2 below −0.7 V RHE compared with Cu NPs/C and SnO 2 NSL/C, revealing that the Cu–SnO 2 bimetallic catalysts are propitious to depress the HER during the CO 2 RR. Moreover, the product FEs of Cu–SnO 2 bimetallic catalysts present a trend as the potentials change from −0.7 to −1.0 V RHE ; FE HCOOH gradually increases along with FE CO and FE H2 decrease, which is different from that of Cu NPs/C or SnO 2 NSL/C, revealing that the combination of Cu and SnO 2 affects the product selectivity of the CO 2 RR. Fig. 3 Electrochemical CO 2 reduction performance of various Cu–SnO 2 catalysts, Cu NPs/C and SnO 2 NSL/C. a Linear sweeping voltammetric curves of electrochemical CO 2 reduction measured in 0.1 M KHCO 3 for different catalysts. Scan rate: 5 mV s −1 . Reduction potential-dependent faradaic efficiencies (FEs) of H 2 , CO, and HCOOH for b CuSn NPs/C-A, c CuSn NPs/C-H, d CuSn NPs/C-AH, e SnO 2 NSL/C, and f Cu NPs/C Full size image To further determine the correlation between CO 2 RR performance and their structures and phases, we summarized the FEs of H 2 , CO, and HCOOH for these five catalysts at −0.7 and −1.0 V RHE in Fig. 4a, b , respectively. It clear shows that the main product of the CO 2 RR was CO under the potential of −0.7 V RHE for CuSn NPs/C-A (70.1% FE CO ) and CuSn NPs/C-AH (45.1% FE CO ), which largely surpassed the CuSn NPs/C-H (20.1% FE CO ), Cu NPs/C (13.5% FE CO ), and SnO 2 NSL/C (8.4% FE CO ). Moreover, at −0.7 V RHE the CuSn NPs/C-A reached the maximum partial current density of CO (1.66 mA cm −2 , Supplementary Fig. 17 ), which was 1.9, 7.9, 5.9, and 33.2 times higher than the values of the CuSn NPs/C-AH (0.86 mA cm −2 ), CuSn NPs/C-H (0.21 mA cm −2 ), Cu NPs/C (0.28 mA cm −2 ), and SnO 2 NSL/C (0.05 mA cm −2 ), respectively (Fig. 4c ). The FE and partial current density for the CO under −0.7 V RHE of the CuSn NPs/C-A surpass the reported oxidized-derived copper catalysts [6] , [33] , [35] , the home-made oxidized-derived copper (CuO NPs/C and Cu 2 O NPs/C catalysts) (Supplementary Fig. 18 and Supplementary Fig. 19 ), and even comparable to those reported Au [8] , Ag [11] , and Pd [12] catalysts. When the potential applied was −1.0 V RHE , the FEs of CO and H 2 sharply decreased, with HCOOH as the main product for all catalysts except for Cu NPs/C. Particularly, the CuSn NPs/C-A still achieved the highest FE HCOOH of 71.5%, successfully realizing the tuning of the product FE from CO to HCOOH at ~70% by simply changing the electrolysis potential. Such tunable selectivity of CO and HCOOH at high levels surpassed most reported Cu-based bimetallic CO 2 RR catalysts (Supplementary Table 1 ). Meanwhile, at −1.0 V RHE the CuSn NPs/C-A also exhibited the highest partial current density of HCOOH (12.6 mA cm −2 , Fig. 4d ), which exceeded the CuSn NPs/C-AH (10.8 mA cm −2 ) and CuSn NPs/C-H (10.5 mA cm −2 ) and was far better than the Cu NPs/C and SnO 2 NSL/C. Finally, the long-term stabilities of CuSn NPs/C-A, CuSn NPs/C-H, and CuSn NPs/C-AH were also investigated using chronoamperometry at −0.7 V RHE . As shown in Supplementary Fig. 20 , all the above catalysts achieved stable current densities in the span of 10 h. Meanwhile, the product FE values of these catalysts could also be maintained at the initial value, suggesting that the CO 2 RR performances of these Cu–SnO 2 bimetallic catalysts is stable. Furthermore, the hollow SnO 2 shell and heterostructure of CuSn NPs/C-A were largely maintained after the stability test, revealing the stable structure of CuSn NPs/C-A (Supplementary Fig. 21 ). Fig. 4 Comparison of the faradaic efficiencies (FEs) and partial current densities of the electrochemical CO 2 reduction products for various catalysts under specific potential. Histograms of CO, H 2 and HCOOH FEs at a −0.7 V RHE and b −1.0 V RHE for different catalysts. Histograms of current densities of c CO at −0.7 V RHE and d HCOOH at −1.0 V RHE for different catalysts Full size image It is generally believed that the chemical state and structure of catalysts would gradually undergo changes during the CO 2 RR process, which can largely determine their ultimate performance. To this end, the TEM images and XPS characterizations of CuSn NPs/C-A, CuSn NPs/C-H, and CuSn NPs/C-AH after the 15 min chronoamperometry test at −0.7 V RHE (denoted as CuSn NPs/C-A-ACP, CuSn NPs/C-H-ACP, and CuSn /C-AH-ACP) were carried out to investigate their evolved surface states and structures. As shown in Fig. 5a , while the CuSn NPs/C-A-ACP still maintained the hollow structure during the CO 2 RR, the lattice fringes measured in the enlarged image are 0.209 and 0.180 nm, corresponding to the Cu (111) and Cu (200) planes, respectively, being consistent with the XRD result (Supplementary Fig. 22a ), suggesting that the oxidized Cu 2+ have been reduced into metallic Cu during the CO 2 RR process (Fig. 5b, c ). The chemical state changes of Cu can also be confirmed by the XPS, where the ratio of Cu 0,1+ /Cu 2+ in the CuSn NPs/C-A-ACP increased to 2.7/1, in contrast with 0 in the CuSn NPs/C-A (Supplementary Fig. 23 ). As opposed to Cu, Sn was still in the form of the amorphous SnO 2 combined with the small composition loss in the CuSn NPs/C-A-ACP (Fig. 5b, c and Supplementary Fig. 24a ). The element mapping further reveals that the amorphous SnO 2 was mixed with Cu in the CuSn NPs/C-A-ACP, which can produce numerous Cu/SnO 2 interfaces (Fig. 5d ). In contrast, the CuSn NPs/C-H-ACP maintains the Cu 41 Sn 11 @SnO 2 core–shell structure of the initial CuSn NPs/C-H with small composition change, as confirmed by the HRTEM image, HAADF EDS elemental mappings, XRD, and EDS results (Fig. 5e–h , Supplementary Fig. 22b , and Supplementary Fig. 24b ), indicating that there are hardly any Cu/SnO 2 interfaces exposed. The structure of CuSn NPs/C-AH-ACP also undergoes a significant change, where the original hollow amorphous SnO 2 shrinks into a solid particle combined with the Cu in the CuSn NPs/C-AH-ACP due to the element corrosion and migration during the CO 2 RR process (Fig. 5i , Supplementary Fig. 22c , and Supplementary Fig. 24c ). The enlarged HRTEM and element mapping images further show that the newly evolved structure of CuSn NPs/C-AH-ACP has a few interface between Cu and SnO 2 (Fig. 5j–l , Supplementary Fig. 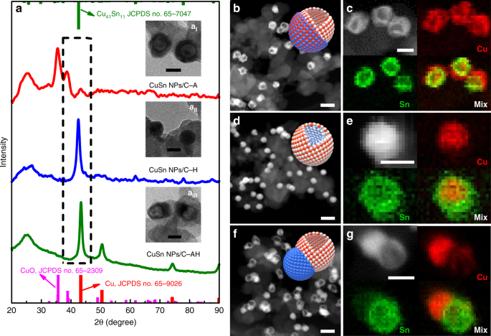25 ). Fig. 2 Structure and phase characterizations of CuSn NPs/C with controlled annealing treatment.aX-ray diffraction (XRD) patterns and inset transmission electron microscopic (TEM) images ofaICuSn NPs/C-A,aIICuSn NPs/C-H, andaIIICuSn NPs/C-AH.b,d,fHigh-angle annular dark-field scanning TEM (HAADF-STEM) images and atom models andc,e,gHAADF-STEM images and energy-dispersive X-ray spectroscopy (EDS) elemental mappings ofb,cCuSn NPs/C-A,d,eCuSn NPs/C-H, andf,gCuSn NPs/C-AH. Scale bars, 50 nm inb,d,f, 20 nm inaI–aIII,c,e,g. Red, blue, and white spheres in the models represent O, Cu, and Sn atoms, respectively Moreover, the surface composition of the above catalysts was also confirmed by XPS results (Supplementary Table 2 ). The ratios of Cu/Sn in CuSn NPs/C-H-ACP and CuSn NPs/C-AH-ACP calculated by the XPS results are lower than those by EDS results, suggesting that the Sn is mainly located on the surface in these catalysts, being consistent with the results of element mapping. Moreover, according to the XPS results the ratio of Cu/Sn in CuSn NPs/C-A-ACP is similar with the CuSn NPs/C-AH-ACP, indicating that the composition effect on the FE CO improvement of CuSn NPs/C-A-ACP and CuSn NPs/C-AH-ACP is negligible. Thus, with the surface state and structure evolutions of different catalysts, the greatest difference among them is the density of the newly formed Cu/SnO 2 interfaces, which follows the sequence: CuSn NPs/C-A-ACP > CuSn NPs/C-AH-ACP > CuSn NPs/C-H-ACP. Therefore, it is reasonable to conclude that the newly produced Cu/SnO 2 interfaces are the active sites for improving the catalytic selectivity in those Cu–SnO 2 bimetallic catalysts and resulting in the different selectivity for the CO 2 RR. To further prove it, the mixed Cu NPs/C and SnO 2 NSL/C with similar Cu/Sn ratio but limited Cu/SnO 2 interfaces were used as the catalyst for the CO 2 RR (Supplementary Fig. 26 ). It is shown that the FE CO of mixed Cu NPs/C and SnO 2 NSL/C at −0.7 V RHE is 31.3% (Supplementary Fig. 27 ), which is between the FE CO of CuSn NPs/C-H and of CuSn NPs/C-AH. Based on the TEM and HRTEM observation and the CO 2 RR results of various catalysts, we can conclude that the FEs CO of different catalysts are systematically controlled by the Cu/SnO 2 interfaces (Supplementary Fig. 28 ), confirming the importance of Cu/SnO 2 interfaces in boosting the product selectivity of CO 2 RR. Fig. 5 Structure and interface characterizations of CuSn NPs/C-A-ACP, CuSn NPs/C-H-ACP, and CuSn NPs/C-AH-ACP. a , e , i High-resolution transmission electron microscopy (HRTEM) images, b , c , f , g , j , k magnified HRTEM images, and d , h , l high-angle annular dark-field scanning TEM (HAADF-STEM) image and energy-dispersive X-ray spectroscopy (EDS) elemental mappings of a – d CuSn NPs/C-A-ACP, e – h CuSn NPs/C-H-ACP, and i – l CuSn NPs/C-AH-ACP. Scale bars, 10 nm in d , h , l , 5 nm in a , e , i , 2 nm in b , c , f , g , j , k Full size image To further elucidate the Cu/SnO 2 interfaces effect on product selectivity for Cu–SnO 2 bimetallic catalysts, the density functional theory (DFT) calculations of Cu–SnO 2 heterostructures were carried out. In general, the CO 2 electroreduction usually initiates with the proton-coupled electron transfer process, then the C or O atom protonation would result in generating OCHO* or COOH* species, respectively. The adsorption free-energies of CO 2 RR intermediates and the Δ G of elementary steps for Cu (111) and SnO 2 (110) surfaces were first calculated employing the computational hydrogen electrode (CHE) model [23] . As shown in Supplementary Fig. 29 , the formation of OCHO* species (Δ G = 0.20 eV) is energetically more favorable than that of COOH* species (Δ G = 0.71 eV) on the Cu (111) surface. Similarly, the SnO 2 (110) surface also favors HCOOH as the final product since the formation of OCHO* (Δ G = 1.48 eV) species is energetically much more favorable than that of COOH*species (Δ G = 2.32 eV) (Supplementary Fig. 30 ). Furthermore, the Cu/SnO 2 interfacial effect on the CO 2 RR electrocatalytic performance of the Cu–SnO 2 heterostructure were explored. 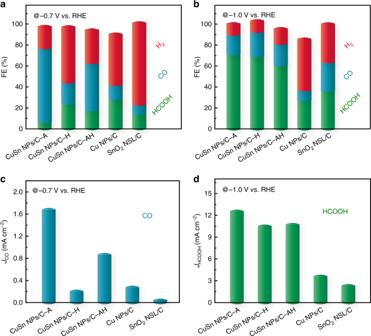Fig. 4 Comparison of the faradaic efficiencies (FEs) and partial current densities of the electrochemical CO2reduction products for various catalysts under specific potential. Histograms of CO, H2and HCOOH FEs ata−0.7 VRHEandb−1.0 VRHEfor different catalysts. Histograms of current densities ofcCO at −0.7 VRHEanddHCOOH at −1.0 VRHEfor different catalysts The Cu/SnO 2 interface was constructed by binding the Sn 6 O 12 cluster onto the Cu (111) slab. Note that the surface-supported small oxide clusters are effective to describe catalytic activity of the complex [36] , [37] . As shown in Fig. 6a , in sharp contrast to individual Cu (111) and SnO 2 (110) surfaces, the O atom rather than the C atom of the CO 2 molecule prefers to be first hydrogenated at the Cu/SnO 2 interface. Specifically, the Δ G for the COOH* species formation is 0.52 eV at Cu/SnO 2 interfaces, being lower than those of 0.71 and 2.32 eV at the Cu (111) surface and SnO 2 (110) surface, respectively. Meanwhile, the COOH* species formation is energetically more favorable than that of OCHO* species (Δ G = 0.85 eV) at Cu/SnO 2 interfaces. The COOH* intermediate can be easily converted to a removed H 2 O molecule and an adsorbed CO* species with a Δ G of 0.43 eV. Finally, the CO* species can be desorbed easily with a ΔG of −0.13 eV to form the CO. The calculations vividly demonstrated that the construction of the Cu/SnO 2 interface can essentially tune the catalytic products and enhance the activity of Cu–SnO 2 bimetallic catalysts to generate CO, which are in good agreement with experimental observations. Thus owing to the more evolved Cu/SnO 2 interfaces than that of the CuSn NPs/C-AH during the CO 2 RR process (Fig. 6b ), the CuSn NPs/C-A shows a higher FE CO at −0.7 V RHE . However, for the CuSn NPs/C-H, the exposed reactive site is only SnO 2 (Fig. 6b ), resulting in both high FE H2 and FE HCOOH values. Although Sarfaz et al. and Li et al. [28] have also shown high FE CO at lower overpotential for CO 2 RR by the CuSn complex structures, the active site for improving the CO 2 RR performance is vague. In fact, the biggest concept difference between our work and Sarfaz’s work/Li’s work is that the Sarfaz’s work/Li’s work mainly focused on controlling the Cu/Sn composition and SnO 2 thickness to tune the CO 2 RR, while the unexplored phase/structure effects of Cu/Sn catalysts for enhancing CO 2 RR have been decoded in our work. This is also the main reason why we can generate both CO and HCOOH with high selectivity, while only high FE CO can be obtained in Sarfaz’ work/Li’s work. 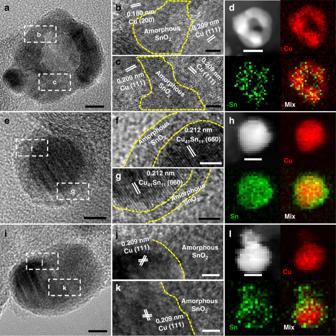Fig. 5 Structure and interface characterizations of CuSn NPs/C-A-ACP, CuSn NPs/C-H-ACP, and CuSn NPs/C-AH-ACP.a,e,iHigh-resolution transmission electron microscopy (HRTEM) images,b,c,f,g,j,kmagnified HRTEM images, andd,h,lhigh-angle annular dark-field scanning TEM (HAADF-STEM) image and energy-dispersive X-ray spectroscopy (EDS) elemental mappings ofa–dCuSn NPs/C-A-ACP,e–hCuSn NPs/C-H-ACP, andi–lCuSn NPs/C-AH-ACP. Scale bars, 10 nm ind,h,l, 5 nm ina,e,i, 2 nm inb,c,f,g,j,k 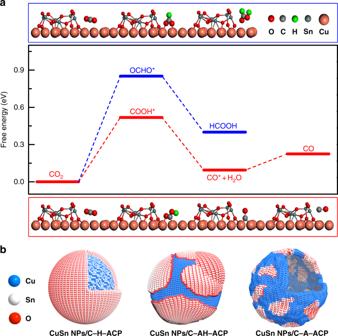Fig. 6 Density functional theory simulations of the CO2reduction reaction on Cu/SnO2interfaces.aFree energy profiles of two pathways for CO2electroreduction on Cu/SnO2interfaces. The upper and lower images are optimized geometric structures of various states (COOH*, OCHO*, and CO*) of the process on Cu/SnO2interfaces, respectively. H, C, O, Cu, and Sn atoms are represented by green, gray, red, reddish brown, and dark gray spheres, respectively.bThe models of CuSn NPs/C-A-ACP, CuSn NPs/C-H-ACP, and CuSn NPs/C-AH-ACP with different Cu/SnO2interfaces By further combining the experimental characterizations with the DFT calculations, we have revealed the important role of Cu/SnO 2 interfaces on enhancing the CO 2 RR, which makes a progress to understand the phase and structure effects for improving the CO 2 RR performance. Fig. 6 Density functional theory simulations of the CO 2 reduction reaction on Cu/SnO 2 interfaces. a Free energy profiles of two pathways for CO 2 electroreduction on Cu/SnO 2 interfaces. The upper and lower images are optimized geometric structures of various states (COOH*, OCHO*, and CO*) of the process on Cu/SnO 2 interfaces, respectively. H, C, O, Cu, and Sn atoms are represented by green, gray, red, reddish brown, and dark gray spheres, respectively. b The models of CuSn NPs/C-A-ACP, CuSn NPs/C-H-ACP, and CuSn NPs/C-AH-ACP with different Cu/SnO 2 interfaces Full size image In summary, by simple thermal annealing of CuSn core–shell NPs in controlled conditions, we have created Cu–SnO 2 catalysts with three distinct engineered structures and phases: the CuO/hollow SnO 2 heterostructure of CuSn NPs/C-A, the Cu 41 Sn 11 @SnO 2 core–shell structure of CuSn NPs/C-H, and the Cu NPs/hollow SnO 2 Janus structure of CuSn NPs/C-AH. Benefitting from the abundant Cu/SnO 2 interfaces involved in the CuO/hollow SnO 2 heterostructure during the electrochemical process, the CuSn NPs/C-A exhibits promising electrocatalytic performance for CO 2 RR due to the decreased Δ G for the formation of COOH* species at Cu/SnO 2 interfaces. It shows the highest activity toward CO 2 RR in all the Cu–SnO 2 heterostructures, with partial current densities of CO at −0.7 V RHE over 5.9 and 5.3 times higher and of HCOOH at −1.0 V RHE over 33.2 and 3.4 times higher than those of the Cu NPs/C and SnO 2 NSL/C, respectively. Particularly, the CuSn NPs/C-A can tune the products from CO to HCOOH with an FE at approximately 70% by simply changing the electrolysis potentials. These Cu–SnO 2 bimetallic catalysts also exhibit excellent durability after the long-term chronoamperometry test at −0.7 V RHE . The present study highlights a phase and structure-engineering strategy for creating high-performance electrocatalysts for the CO 2 RR and beyond. Chemicals Copper (II) acetylacetonate (Cu(acac) 2 , 97%), AA (AR), and oleylamine (CH 3 (CH 2 ) 7 CH=CH(CH 2 ) 7 CH 2 NH 2 , 70%) were all purchased from Sigma-Aldrich. Potassium bicarbonate (KHCO 3 , AR) was purchased from Sinopharm Chemical Reagent Co. Ltd. (Shanghai, China). Dibutyltin bis(2,4-pentanedionate) (C 18 H 32 O 4 Sn) was purchased from Strem Chemical. Nitrogen (N 2 , 99.999%) and carbon dioxide (CO 2 , 99.999%) were purchased from WuGang Gas Co. Ltd. (Shanghai, China). All the above chemicals were directly used without further purification. The water (18 MΩ*cm) used in all experiments was prepared with an ultra-pure purification system. Preparation of CuSn NPs In a typical preparation of CuSn NPs, 13.3 mg Cu(acac) 2 , 6 μL C 18 H 32 O 4 Sn, 27 mg AA, and 5 mL oleylamine were mixed and ultrasonicated for approximately 0.5 h in a sealed vial (30 mL). Then the vial was transferred into an oil bath and heated at 180 °C for 3 h. The resulting colloidal products in the vial were collected by centrifugation and washed with an ethanol/cyclohexane mixture to obtain CuSn NPs. Preparation of CuSn NPs/C, CuSn NPs/C-A, CuSn NPs/C-H, and CuSn NPs/C-AH In a typical preparation of CuSn NPs/C, CuSn NPs were mixed with VC-X72 carbon in 10 mL cyclohexane and sonicated for 1 h to deposit them on carbon. The products were separated by centrifugation and washed with cyclohexane/ethanol to generate CuSn NPs/C. The CuSn NPs/C was annealed in air at 250 °C for 1 h and 5% H 2 +95% N 2 mixed gas at 250 °C for 1 h to obtain CuSn NPs/C-A and CuSn NPs/C-H, respectively. The CuSn NPs/C-A sample was further annealed in 5% H 2 +95% N 2 at 250 °C for another 1 h to generate CuSn NPs/C-AH. The mass loadings in all the catalysts were fixed to be 10%+0.5%, as analyzed by inductively coupled plasma atomic emission spectroscopy (ICP-AES). Preparation of Cu NPs and Cu NPs/C The preparation of Cu NPs was similar to that of CuSn NPs but without adding C 18 H 32 O 4 Sn. The resulting products were collected by centrifugation and washed with an ethanol/cyclohexane mixture. The obtained Cu NPs were then mixed with VC-X72 carbon in 10 mL cyclohexane and sonicated for 1 h to deposit them on carbon. The products were separated by centrifugation and washed with cyclohexane/ethanol to generate Cu NPs/C. Preparation of SnO 2 NSL/C In a typical preparation of SnO 2 NSL/C, 10 mg CuSn NPs/C-A were mixed with 8 mL ethanol and 2 mL acetic acid and ultrasonicated for 1 h to remove the CuO. The products were separated by centrifugation and washed with ethanol to generate SnO 2 NSL/C. Characterization TEM and HAADF-STEM were conducted on an FEI Tecnai F20 transmission electron microscope with acceleration voltage of 200 kV. The samples were prepared by dropping samples dispersed in cyclohexane or ethanol onto carbon-coated copper TEM grids using pipettes and were dried under ambient conditions. XRD patterns were collected on the X’Pert-Pro MPD diffractometer (Netherlands PANalytical) with a Cu Kα X-ray source ( λ = 1.540598 Å). The concentrations of catalysts were determined by ICP-AES (710-ES, Varian). XPS was performed with an SSI S-Probe XPS Spectrometer. The carbon peak at 284.6 eV was used as a reference to correct for charging effects. Electrochemical measurements The electrochemical measurements of CO 2 RR was performed by a three-electrode system with a carbon paper (Toray, 1 × 1 cm 2 ) as working electrode, a micro Ag/AgCl electrode (4.0 M KCl) as reference electrode, and a Pt wire as the reference electrode. In the preparation of working electrode, 8 mg catalyst was ultrasonicated with 380 µL of ethanol, 20 µL of water, and 5 µL of a 5 wt% Nafion solution for 1 has catalyst ink. Then 100 µL of the catalyst ink was dropped onto carbon paper and aired to obtain the working electrodes. The electrochemical measurements was conducted in an H-cell reactor with an anion exchange membrane (Nafion 117) on CHI660 (Chenhua, Shanghai) electrochemical workstation. Each chamber of the H-cell contained 60 mL of 0.1 M KHCO 3 aqueous solution with an ~40 mL headspace. For the electrochemical measurements, the CO 2 was delivered into the cathodic compartment (directly connected to the gas chromatograph (GC Agilent 7890B)) at a constant rate of 20 sccm and was allowed to purge for 30 min prior to the beginning of experiments. The gas-phase composition was analyzed by a GC equipped with a PLOT MolSieve 5A column and a Q-bond PLOT column every 15 min with different potentials applied. Liquid products were analyzed by 1 H NMR on Agilent 600 MHz DirectDrive2 spectrometers. All potentials were given against the reversible hydrogen electrode (RHE), calculated using the Nernst equation, and the readouts were recorded with 90% Ohmic iR drop correction. The FE for the products was calculated as follows: 
    FE = eF× n/Q
 (1) where e is the number of electrons transferred for different products, Q is the total charge, n is the total amount of different product (in moles), and F is the Faraday constant. Computational method DFT calculations were performed using the plane-wave technique implemented in the Vienna ab initio simulation package [38] , [39] . The ion–electron interaction was described using the projector-augmented plane wave approach [40] . The generalized gradient approximation expressed by the Perdew–Burke–Ernzerhof functional [41] and a 360-eV cutoff for the plane-wave basis set were adopted in all the computations. To simulate the Cu/SnO 2 interfaces, we placed a Sn 6 O 12 cluster on a 5×5×3 Cu (111) surface with a 19-Å vacuum between the slabs. The Sn 6 O 12 cluster was built based on rutile SnO 2 bulk crystal and resembles the SnO 2 (110) surface structure. For comparison, a 4×4×3 Cu (111) slab with a 3×3×1 k -point sampling was used. The SnO 2 (110) surface was modeled by a six atomic layer, and the top three atomic layers were relaxed while the other layers were fixed at the bulk lattice position. For Cu–SnO 2 and the Cu (111) slab, the upper most layer (including the Cu (111) slab and Sn 6 O 12 cluster) were allowed to relax, except for those of the bottom two layers in Cu (111), which were fixed at the bulk lattice position. The Gaussian smearing method with σ value of 0.1 eV was used in this system. The convergence threshold was set as 10 −4 eV in energy and 0.08 eV Å −1 in force. A (2 × 2 × 1) gamma centered k -point was chosen for the slab calculation. The solvent effect on adsorbates was simulated using the Poissson–Boltzmann implicit solvation model with a dielectric constant of 80 [42] . The effects of dipole correction for adsorbates were also included. The CHE method has been applied to determine the Gibbs free energy of the reaction species. In this method, the electrochemical potential of an electron–proton pair (H + + e − ) is equal to the free energy of half of hydrogen (1/2 H 2 ) at standard pressure. The CO 2 RR involving a 2 e pathway can be described by: 
    CO_2( g) + ( H^ + + e^ - ) + ∗→OCHO∗
 (2) 
    OCHO^∗ + ( H^ + + e^ - ) →∗ + HCOOH( l)
 (3) 
    CO_2( g) + ( H^ + + e^ - ) + ∗→COOH∗
 (4) 
    COOH∗ + ( H^ + + e^ - ) →CO∗ + H_2O→∗ + CO( g)
 (5) where * represents the adsorption site, while OCHO*, COOH*, and CO* represent reaction intermediates, respectively. The free energy ( G ) of each intermediate estimated at T = 298 K was expressed as: 
    G = E_DFT + E_ZPE - TS +  C_pdT
 (6) where E DFT , E ZPE , S , and C p were the electronic energy, zero point energy, entropy, and heat capacity, respectively. For adsorbed intermediates, E ZPE , S , and C p were determined by vibration frequency calculations via standard methods, where all 3 N degrees of freedom were treated as harmonic vibration motions with neglecting contributions from the slab; for molecules, however, those values were taken from the NIST database [43] . The contribution of zero point energy, entropy corrections, and heat capacity to G is provided in Supplementary Table 3 .